Bit-by-bit autophagic removal of parkin-labelled mitochondria Eukaryotic cells maintain mitochondrial integrity through mitophagy, an autophagic process by which dysfunctional mitochondria are selectively sequestered into double-layered membrane structures, termed phagophores, and delivered to lysosomes for degradation. Here we show that small fragments of parkin-labelled mitochondria at omegasome-marked sites are engulfed by autophagic membranes one at a time. Using a light-activation scheme to impair long mitochondrial tubules, we demonstrate that sites undergoing bit-by-bit mitophagy display preferential ubiquitination, and are situated where parkin-labelled mitochondrial tubules and endoplasmic reticulum intersect. Our observations suggest contact regions between the endoplasmic reticulum and impaired mitochondria are initiation sites for local LC3 recruitment and mitochondrial remodelling that support bit-by-bit, parkin-mediated mitophagy. These results help in understanding how cells manage to fit large and morphologically heterogeneous mitochondria into micron-sized autophagic membranes during mitophagy. Eukaryotic cells maintain mitochondrial integrity through an autophagic process termed mitophagy [1] , [2] , [3] ; dysfunctional mitochondria are selectively sequestered into double-layered membrane structures termed phagophores and are delivered to lysosomes for degradation. The importance of this process is best exemplified by the fact that two proteins found mutated in autosomal recessive forms of Parkinson’s disease, parkin and PINK1 (phosphatase and tensin homologue-induced putative kinase protein 1), have central roles in this process, connecting mitophagy dysfunction to Parkinsonism [4] , [5] . PINK1 senses mitochondrial impairment and recruits parkin, a ubiquitin E3 ligase, from the cytoplasm onto dysfunctional mitochondria [6] , [7] , [8] , [9] , [10] . The parkin-decorated mitochondrial tubules then become substrates for mitophagic turnover. A cell needs to encase these large and morphologically heterogeneous parkin-labelled mitochondria into autophagic membranes for the proper progression of mitophagy. Here, by light-impairing long mitochondrial tubules, we found that they became autophagocytosed one fraction at a time. These actions took place preferentially at omegasome-marked endoplasmic reticulum (ER) subdomains, requiring proteasome-mediated mitochondrial remodelling. We suggest ER/impaired mitochondria contact regions as initiation platforms for bit-by-bit, parkin-mediated mitophagy. Observation of bit-by-bit mitophagy The autophagic machinery needs to be able to turn over impaired mitochondrial tubules to avoid the accumulation of damaged mitochondria, a condition that has been implicated in Parkinson’s disease. Dimensions of typical phagophores and the resulting autophagosomes in mammalian cells range only between a few hundred nanometres to a micron, and can be slightly expanded under conditions when autophagy is activated (such as during starvation) [11] . Such sizes can be too small for the engulfment of mitochondrial tubules during mitophagy. As can be seen in Fig. 1a with HeLa cell expressing EGFP-LC3, the length of mitochondrial tubules, as stained by tetramethylrhodamine ethyl ester (TMRE), can run over several microns, whereas the LC3-marked autophagosomes are sub-micron-sized. The LC3 puncta in HeLa cells remained in the single-micron range even during starvation (right panel, Fig. 1a ). We therefore aimed to investigate how impaired mitochondrial tubules get packaged into smaller-sized LC3 structures during mitophagy. 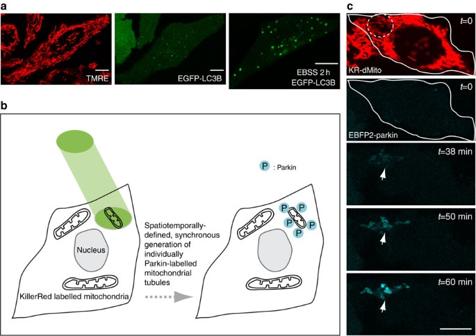Figure 1: Generating defined parkin-labelled mitochondria as substrates for autophagy. (a) Mitochondrial tubules in HeLa cells (top, TMRE stained) exceeded the dimensions of that for autophagosomes (labelled by EGFP-LC3B) under either normal (middle, same field as TMRE image) or starvation conditions (right). (b) Diagram of light-induced mitophagy. Single mitochondrial tubules containing KR-dMito, when illuminated by 559 nm light, are selectively impaired, leading to surface recruitment of parkin and subsequent autophagic turnover. (c) Illuminating a selective region (white dotted circle, top) within a KR-dMito/EBFP2-parkin-expressing HeLa cell led to the immediate loss of KR fluorescence (top two panels). Third to fifth row: magnified view of the photo-impaired region, EBFP2-parkin translocated onto impaired mitochondrial tubules synchronously (38–60 min after 559 illumination, white arrows). Scale bars (all panels), 10 μm. Figure 1: Generating defined parkin-labelled mitochondria as substrates for autophagy. ( a ) Mitochondrial tubules in HeLa cells (top, TMRE stained) exceeded the dimensions of that for autophagosomes (labelled by EGFP-LC3B) under either normal (middle, same field as TMRE image) or starvation conditions (right). ( b ) Diagram of light-induced mitophagy. Single mitochondrial tubules containing KR-dMito, when illuminated by 559 nm light, are selectively impaired, leading to surface recruitment of parkin and subsequent autophagic turnover. ( c ) Illuminating a selective region (white dotted circle, top) within a KR-dMito/EBFP2-parkin-expressing HeLa cell led to the immediate loss of KR fluorescence (top two panels). Third to fifth row: magnified view of the photo-impaired region, EBFP2-parkin translocated onto impaired mitochondrial tubules synchronously (38–60 min after 559 illumination, white arrows). Scale bars (all panels), 10 μm. Full size image Mitochondrial tubules can be impaired and targeted for parkin-mediated mitophagy with spatial and temporal precision using light illumination [12] ( Fig. 1b ). In HeLa cells expressing mitochondria-targeted photosensitizer KillerRed [13] (KR-dMito) and EBFP2-parkin, one can utilize 559 nm illumination to selectively photo-inactivate mitochondria. Exciting KillerRed with 559 nm light led to spatiotemporally defined reactive oxygen species (ROS) generation within the mitochondrial matrix, which caused immediate mitochondrial impairment and elicited synchronous recruitment of parkin onto specific mitochondria within the light-illuminated region ( Fig. 1c ). This allowed us to control the dimensions of parkin-labelled mitochondria precisely with light and to probe how cell encapsulate large mitochondrial tubules into LC3-coated autophagic structures during mitophagy [14] . To enable clear visualization of mitophagy, we illuminated areas displaying sparse mitochondrial networks in HeLa cells expressing KR-dMito, EGFP-LC3B and EBFP2-parkin ( Fig. 2a ). Mitochondria targeted by this tightly controlled operation underwent parkin-mediated mitophagy but was able to maintain their original tubular morphology even after parkin had uniformly and synchronously coated the entire mitochondrial outer membrane ( Fig. 2b , white arrows; parkin uniformly and synchronously covered all areas of the photo-impaired mitochondria). Our parkin-labelled mitochondrial tubules preserved the ability to undergo active transport, as well as fusion and fission ( Supplementary Fig. S1 and Supplementary Movie 1 ). The individual parkin-labelled tubule generated is well beyond the dimension of autophagic structures normally seen in HeLa cells. Although the entire mitochondrial tubule was photo-impaired at once, as was parkin recruitment ( Supplementary Movie 2 ), the subsequent engulfment into autophagosomes, however, was not. Instead of being engulfed into a single long LC3-coated autophagic structure, multiple small but discrete autophagosomes formed along the parkin-labelled tubule ( Fig. 2c ). The observed LC3 spots on the impaired mitochondria possessed characteristic sizes resembling that of normal autophagosomes. These individual LC3-coated autophagic structures then one-by-one trafficked away fractions of the parkin-labelled mitochondria for removal ( Fig. 2d ; in some instances, multiple LC3/parkin spot fused into a larger puncta during trafficking, Supplementary Fig. S2 ). The fact that the single parkin-labelled mitochondria tubule needed to be engulfed in a bit-by-bit fashion through LC3 structures is in accordance with our observation that the parkin-labelled tubule gradually fragmented into multiple smaller pieces ( Supplementary Movie 3 ). Two modes of autophagic engulfment for photo-impaired mitochondria were observed: sub-micron-sized parkin-labelled mitochondria particles were engulfed as a whole, with LC3 nucleated on single locations along these structures, and subsequently wrapped around the entire particles ( Supplementary Fig. S3a ). In contrast, tubules of a few microns in length displayed step-by-step clearance through autophagy, with LC3 structures asynchronously nucleating on multiple distinct locations on the tubules to carry out mitophagy ( Supplementary Fig. S3b ). 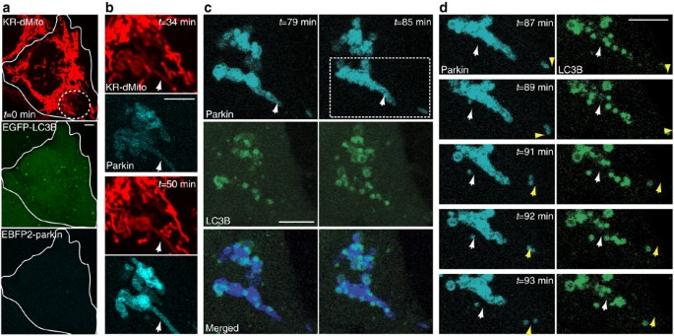Figure 2: Bit-by-bit removal of parkin-labelled mitochondria by autophagy. (a) A HeLa cell expressing KR-dMito, EGFP-LC3B and EBFP2-parkin (cyan) were 559 nm illuminated (white dotted circle region; immediate loss of KR fluorescence). (b–d) Magnified view of the photo-inactivated region ina34–93 min after 559 nm illumination. (b) Induction of parkin-mediated mitophagy on a single, long mitochondria tubule (white arrows). (c) LC3B-coated structures were recruited onto distinct spots on the photo-impaired mitochondrial tubule (white arrows: the location of the original impaired single mitochondrial tubule). (d) White dotted line region outlined inc, LC3 structures segregated from the main parkin-labelled cluster, carrying away bits of the parkin-labelled mitochondria with them. Two individual events are labelled in the image sequence with white and yellow arrows, respectively. Scale bars (all panels), 5 μm. Figure 2: Bit-by-bit removal of parkin-labelled mitochondria by autophagy. ( a ) A HeLa cell expressing KR-dMito, EGFP-LC3B and EBFP2-parkin (cyan) were 559 nm illuminated (white dotted circle region; immediate loss of KR fluorescence). ( b – d ) Magnified view of the photo-inactivated region in a 34–93 min after 559 nm illumination. ( b ) Induction of parkin-mediated mitophagy on a single, long mitochondria tubule (white arrows). ( c ) LC3B-coated structures were recruited onto distinct spots on the photo-impaired mitochondrial tubule (white arrows: the location of the original impaired single mitochondrial tubule). ( d ) White dotted line region outlined in c , LC3 structures segregated from the main parkin-labelled cluster, carrying away bits of the parkin-labelled mitochondria with them. Two individual events are labelled in the image sequence with white and yellow arrows, respectively. Scale bars (all panels), 5 μm. Full size image ER-associated omegasomes in bit-by-bit mitophagy The fact that impaired mitochondria were processed through autophagy in a bit-by-bit fashion were further evidenced by the observation that pre-autophagosomal structures, such as omegasomes, accumulated focally along parkin-labelled mitochondrial tubules. Past studies in mammalian cells have demonstrated that LC3-marked autophagic structures can emerge from omegasomes (proposed to originate either from the ER [15] , [16] or the ER–mitochondria contact sites [17] ). The molecular marker double FYVE containing protein 1 (DFCP1) labels omegasomes and has been visualized to localize onto damaged mitochondria [15] , [16] , [18] , and was therefore used to visualize the early stages of autophagic membrane generation for engulfing impaired mitochondrial tubules. We photogenerated a single, long parkin-labelled mitochondria for turnover within a HeLa cell co-expressing KR-dMito, EGFP-DFCP1 and EBFP2-parkin (white arrow, Fig. 3a ). Remarkably, EGFP-DFCP1-coated omegasomes formed along the parkin-labelled mitochondria at discrete spots, reminiscent of LC3 actions (white arrows, Fig. 3b ). The focal appearance of DFCP1 along mitochondrial tubules was specific for mitophagy, as omegasomes did not selectively target mitochondria during starvation-induced autophagy ( Supplementary Fig. S4 ). Furthermore, the DFCP1 puncta observed on the impaired mitochondria were highly transient in nature (white arrows, Fig. 3c ). This implied that omegasomes dynamically formed at distinct sites on impaired mitochondrial tubules to initiate LC3 structure generation for bit-by-bit engulfment of mitochondria during parkin-mediated mitophagy. Through imaging carbonyl cyanide 3-chlorophenylhydrazone [7] (CCCP, a mitochondria membrane potential disrupter)-treated COS-7 cells (in which the ER network can be clearly resolved through confocal microscopy) co-expressing EBFP2-parkin, AcGFP-sec61β and TagRFP-DFCP1 undergoing mitophagy, we, in addition, found that omegasomes arose selectively at regions where ER(sec61β) [19] and parkin-labelled mitochondria were spatially associated ( Fig. 3d ). These observations together suggest that ‘contact’ between ER and impaired mitochondria as initiation platforms for our observed bit-by-bit mitophagic actions. 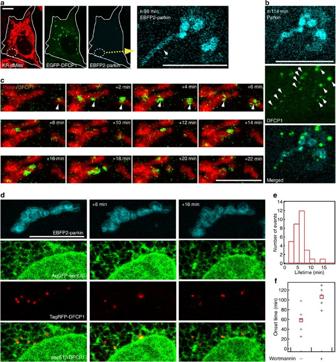Figure 3: Omegasomes form where ER and parkin-labelled mitochondria overlap. (a) A HeLa cell expressing KR-dMito (red), EGFP-DFCP1 (green) and EBFP2-parkin (cyan) were illuminated with 559 nm at the white dotted circle region, leading to the generation of a long parkin-labelled mitochondria tubule (right, magnified view of the light-activated region) for autophagic turnover (white arrow). Scale bars, 10 μm. (b) After the generation of parkin-labelled mitochondrial tubules following treatments ina, discrete DFCP1 foci (green, middle panel, ER-associated omegasomes) formed along the parkin-labelled mitochondria (white arrows indicate DFCP1 spots that colocalized with parkin). Bottom panel: merged image of parkin and DFCP1. Scale bar, 10 μm. (c) Time-lapse imaging showing DCFP1 puncta formation on parkin-labelled mitochondria. A HeLa cell expressing KR-dMito, EGFP-DFCP1 (green) and EBFP2-parkin (pseudo-coloured red) were 559 nm illuminated, leading to the generation of parkin-labelled mitochondria tubules. Time-lapse imaging (1 frame per min) revealed that DFCP1 puncta (green) formed transiently at discrete sites on parkin-labelled mitochondrial tubules (red). White arrows mark two DFCP1 puncta (ER-associated omegasomes) formation/disassembly events directly on parkin-labelled tubules. Scale bar, 5 μm. (d) A COS-7 cell expressing EBFP2-parkin (cyan), AcGFP-sec61β (green) and TagRFP-DFCP1 (red) were treated with 10 μM CCCP for 4 h and imaged. Omegasomes (DFCP1) appeared where ER (sec61β) and impaired mitochondria (parkin) overlap. Scale bar, 10 μm. (e) Histogram of the lifetime of individual DFCP1 foci on parkin-labelled mitochondria in CCCP-treated HeLa cells expressing TagRFP-DFCP1, EGFP-LC3B and EBFP2-parkin. (f) Wortmannin treatments delayed the initial LC3 recruitment times onto parkin-labelled mitochondria in HeLa cells expressing KR-dMito, EGFP-LC3B and EBFP2-parkin. Each ‘+’ marks the times measured in individual HeLa cells (the red ‘□’ (square) denotes the average from five cells).P=0.0172 (Student’st-test). Figure 3: Omegasomes form where ER and parkin-labelled mitochondria overlap. ( a ) A HeLa cell expressing KR-dMito (red), EGFP-DFCP1 (green) and EBFP2-parkin (cyan) were illuminated with 559 nm at the white dotted circle region, leading to the generation of a long parkin-labelled mitochondria tubule (right, magnified view of the light-activated region) for autophagic turnover (white arrow). Scale bars, 10 μm. ( b ) After the generation of parkin-labelled mitochondrial tubules following treatments in a , discrete DFCP1 foci (green, middle panel, ER-associated omegasomes) formed along the parkin-labelled mitochondria (white arrows indicate DFCP1 spots that colocalized with parkin). Bottom panel: merged image of parkin and DFCP1. Scale bar, 10 μm. ( c ) Time-lapse imaging showing DCFP1 puncta formation on parkin-labelled mitochondria. A HeLa cell expressing KR-dMito, EGFP-DFCP1 (green) and EBFP2-parkin (pseudo-coloured red) were 559 nm illuminated, leading to the generation of parkin-labelled mitochondria tubules. Time-lapse imaging (1 frame per min) revealed that DFCP1 puncta (green) formed transiently at discrete sites on parkin-labelled mitochondrial tubules (red). White arrows mark two DFCP1 puncta (ER-associated omegasomes) formation/disassembly events directly on parkin-labelled tubules. Scale bar, 5 μm. ( d ) A COS-7 cell expressing EBFP2-parkin (cyan), AcGFP-sec61β (green) and TagRFP-DFCP1 (red) were treated with 10 μM CCCP for 4 h and imaged. Omegasomes (DFCP1) appeared where ER (sec61β) and impaired mitochondria (parkin) overlap. Scale bar, 10 μm. ( e ) Histogram of the lifetime of individual DFCP1 foci on parkin-labelled mitochondria in CCCP-treated HeLa cells expressing TagRFP-DFCP1, EGFP-LC3B and EBFP2-parkin. ( f ) Wortmannin treatments delayed the initial LC3 recruitment times onto parkin-labelled mitochondria in HeLa cells expressing KR-dMito, EGFP-LC3B and EBFP2-parkin. Each ‘+’ marks the times measured in individual HeLa cells (the red ‘□’ (square) denotes the average from five cells). P =0.0172 (Student’s t -test). Full size image We therefore explored whether discrete ER-associated omegasomes observed on parkin-labelled mitochondria were directly responsible for the generation of individual LC3-labelled autophagic structures that carried out bit-by-bit mitophagic actions. To do this, we followed parkin-mediated mitophagy in CCCP-treated HeLa cells co-expressing TagRFP-DFCP1, EGFP-LC3B and EBFP2-parkin. CCCP treatment led to the formation of clustered, perinuclear-localized parkin-labelled mitochondria as previously reported ( Supplementary Fig. S5a ) [7] . LC3B and DFCP1 colocalized at discrete locations on the parkin-labelled mitochondria ( Supplementary Fig. S5a ). Furthermore, time-lapse imaging revealed that LC3 structures indeed originated from omegasomes residing on parkin-mitochondria (white asterisks and double asterisks, Supplementary Fig. S5b ; greater than 85% of the LC3 spots can be assigned to have originated from transient DFCP1 foci using a 1 min per frame imaging rate): DFCP1-labelled omegasomes first nucleated at distinct sites on parkin-labelled mitochondria, followed by the appearance of LC3-labelled structures at the same locations. DFCP1 signal then disappeared (indicating the disassembly of omegasomes), leaving behind individual LC3-coated autophagic structures on parkin-labelled mitochondria. The mean DFCP1–omegasome lifetime on parkin-labelled mitochondria was between 5 and 6 min, during which defined-sized autophagosomes were generated to locally engulf fractions of parkin-labelled mitochondria for mitophagy ( Fig. 3e ). On the other hand, using a phosphoinositide 3-kinase complex inhibitor wortmannin to reduce omegasome formation significantly delayed the appearance of LC3 structures on parkin-labelled mitochondria ( Fig. 3f ; percentage of parkin-labelled mitochondria covered by LC3 signals 2 h after light activation: 23% with wortmannin, 57% without wortmannin). Collectively, these observations suggested a pivotal role for ER-associated omegasomes in parkin-mediated mitophagy. Focally ubiquitinated regions initiate bit-by-bit mitophagy Next we examined the spatial mitochondrial ubiquitination patterns responsible for encoding bit-by-bit mitophagy. It has been demonstrated that mitochondrial ubiquitination is critical for the proper progression of parkin-mediated mitophagy. During mitophagy, mitochondrial outer membrane proteins, such as voltage-dependent anion channel 1 (VDAC1) become ubiquitinated (mediated by ubiquitin ligases, such as parkin) and attract p62/NDP1 (refs 8 , 10 , 18 , 19 , 20 ), which are adaptor proteins that facilitate mitochondrial clearance through autophagy [20] , [21] , [22] . In CCCP-treated COS-7 cells co-expressing EBFP2-Ub (ubiquitin), AcGFP-sec61β and mcherry-parkin, we observed that although there was global ubiquitination along the entire parkin-labelled mitochondria, distinct foci displaying preferential ubiquitination occurred at sites where ER and impaired mitochondria overlapped ( Fig. 4a , white arrows). This type of ubiquitin foci were similarly observed when we photo-induced mitophagy in HeLa cells co-expressing EBFP2-parkin, EGFP-Ub (ubiquitin) and KR-dMito ( Supplementary Fig. S6 and Supplementary Movie 4 ). Interestingly, VDAC1, a protein known to enrich at ER–mitochondria contact sites [23] , [24] , were also located at these ubiquitin foci ( Supplementary Fig. S7 ). This prompted us to examine whether the mitochondrial-resident ubiquitin foci marked sites for bit-by-bit mitophagy. Through activating mitophagy in HeLa cells co-expressing EBFP2-parkin, EGFP-LC3 and KR-dMito, and post-stained with an anti-ubiquitin antibody ( Fig. 4b ), we found that indeed LC3 structures selectively formed at the ubiquitin foci on parkin-labelled mitochondria ( Fig. 4c , white arrows). DFCP1-labelled omegasomes similarly arose near these ubiquitin foci during mitophagy ( Supplementary Fig. S8 ). These observations further the notion that bit-by-bit mitophagy initiates at the juxtaposition of ER and parkin-labelled mitochondria. 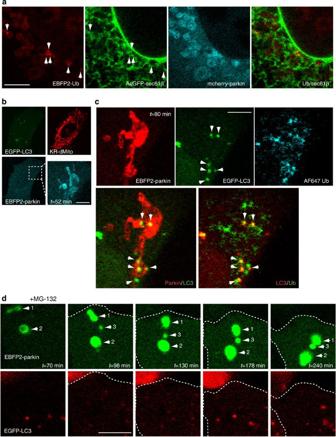Figure 4: Preferentially ubiquitinated foci signal bit-by-bit mitophagy. (a) A COS-7 cell expressing EBFP2-Ub (red), AcGFP-sec61β (green) and mcherry-parkin (cyan) was treated with 10 μM CCCP for 1 h and imaged. Impaired mitochondria (parkin) displayed preferentially ubiquitinated foci (white arrows) at selected regions that overlap with the ER (sec61β). (b) HeLa cells expressing KR-dMito (red), EGFP-LC3 (green) and EBFP2-parkin (cyan) were illuminated with 559 nm at the white dotted square regions, generating parkin-labelled mitochondria (bottom right, magnified view of the light-activated regions). (c) Magnified view of the photo-inactivated region inb80 min after illumination (post-stained with anti-ubiquitin antibody). LC3 and ubiquitin colocalized at discrete sites along parkin-labelled mitochondria (white arrows). (d) A MG-132 treated HeLa cell expressing KR-dMito, EBFP2-parkin (green) and EGFP-LC3B (red) was 559 nm illuminated, leading to the appearance of parkin-labelled mitochondria (white arrows one to three indicated structures, top panels). The parkin-labelled structures did not fragment nor became engulfed by LC3 structures (bottom panels) in the presence MG-132. Scale bars (all panels), 5 μm. Figure 4: Preferentially ubiquitinated foci signal bit-by-bit mitophagy. ( a ) A COS-7 cell expressing EBFP2-Ub (red), AcGFP-sec61β (green) and mcherry-parkin (cyan) was treated with 10 μM CCCP for 1 h and imaged. Impaired mitochondria (parkin) displayed preferentially ubiquitinated foci (white arrows) at selected regions that overlap with the ER (sec61β). ( b ) HeLa cells expressing KR-dMito (red), EGFP-LC3 (green) and EBFP2-parkin (cyan) were illuminated with 559 nm at the white dotted square regions, generating parkin-labelled mitochondria (bottom right, magnified view of the light-activated regions). ( c ) Magnified view of the photo-inactivated region in b 80 min after illumination (post-stained with anti-ubiquitin antibody). LC3 and ubiquitin colocalized at discrete sites along parkin-labelled mitochondria (white arrows). ( d ) A MG-132 treated HeLa cell expressing KR-dMito, EBFP2-parkin (green) and EGFP-LC3B (red) was 559 nm illuminated, leading to the appearance of parkin-labelled mitochondria (white arrows one to three indicated structures, top panels). The parkin-labelled structures did not fragment nor became engulfed by LC3 structures (bottom panels) in the presence MG-132. Scale bars (all panels), 5 μm. Full size image Ubiquitin–proteasome system drives mitochondrial remodelling for bit-by-bit mitophagy We also found mitochondrial ubiquitination to be critical for the proper downsizing/fragmentation of impaired mitochondria for engulfment by autophagosomes. It is now known that aside from LC3 recruitment, ubiquitination mediates mitochondrial protein remodelling and facilitates the rupture of the mitochondrial outer membrane through proteasomal actions during mitophagy [25] , [26] . For example, mitofusin-1 and mitofusin-2 (Mfn2), proteins that drive mitochondrial fusion, are among the most rapidly degraded proteins by the proteasome during mitophagy [25] . In our experiments, inhibition of the ubiquitin–proteasome system function through MG-132 treatment blocked the focal appearance of LC3 structures on parkin-labelled mitochondria ( Fig. 4d ; focal ubiquitination was not affected by MG-132: Supplementary Fig. S9 ). Furthermore, impaired mitochondria tubules became resistant to fragmentation and remained unprocessed by autophagy, leading to the formation large parkin-labelled mitochondrial clusters ( Fig. 4d ). When directly visualizing Mfn2 degradation during mitophagy in HeLa cells co-expressing EBFP2-parkin, EGFP-LC3 and KR-dMito, and post-stained with an anti-Mfn2 antibody ( Supplementary Figs S10a and S11 ), we found parkin-labelled mitochondrial tubules became largely devoid of Mfn2 before focally acquiring LC3 signals ( Supplementary Fig. S10b ). On the contrary, the degradation of Tom20 (a separate proteasome substrate during parkin-mediated mitophagy [25] ) did not precede the appearance of LC3 structures on impaired mitochondria ( Supplementary Fig. S12 ). The lack of Mfn2 along LC3-associated regions on parkin-labelled mitochondria, together with previous reports that Drp1 (dynamin-related protein 1; a mitochondrial fission protein) translocates onto damaged mitochondria [25] , [27] , may allow impaired tubules to be in a pro-fission status to undergo proper downsizing for bit-by-bit mitophagy. Indeed, Drp1 inhibition through mdivi-1 treatments [28] blocked parkin-labelled mitochondria fragmentation ( Supplementary Fig. S13 ). On the other hand, Drp1 could be detected along the entire length of impaired mitochondrial tubules, further suggesting the pro-fission status of parkin-labelled mitochondria ( Supplementary Fig. S14 ). The ubiquitin–proteasome system actions therefore contributed to the dynamic remodelling of impaired mitochondria necessary for mitophagy. Our observations suggested that mitochondria, which are larger than the dimensions of individual autophagosomes, can be cleared through autophagy in a bit-by-bit manner: a fraction of an impaired mitochondrial tubule is packaged into an individual LC3-coated autophagic structure at a time. Although it is currently unknown why global parkin recruitment can lead to focal ubiquitination of impaired mitochondrial tubules, these distinct ubiquitin foci situated at the overlapping regions between ER and parkin-labelled mitochondria serve as initiation sites for omegasome generation and the eventual bit-by-bit autophagic actions. The autophagic machinery is a major materials degradation platform in eukaryotic systems, and is faced with the challenge to turn over a heterogeneous group of cellular materials. Besides mitochondria, many of the substrates are organelles that are also larger than the size of autophagosomes. It will be interesting to find out whether other large cellular structures are also turned over by autophagy in a bit-by-bit fashion similar to that observed on impaired mitochondria during parkin-mediated mitophagy. Plasmids and antibodies EBFP2-parkin was generated by subcloning EBFP2 (Addgene plasmid 14,893) [29] into the EYFP-parkin vector obtained from Addgene (plasmid 23,955) [7] . KillerRed-dMito was purchased from Evrogen (FP964). EGFP-DFCP1, EGFP-VDAC1 and TagRFP-DFCP1 were constructed through PCR amplification of human genes from HeLa cell total complementary DNA, followed by their insertion into EGFP-C1 or pTagRFP-C1 (Evrogen, FP141). EGFP-Ub, AcGFP-sec61β, mcherry-parkin and EGFP-LC3B were obtained from Addgene (plasmids 11,928, 15,108, 23,956 and 11,546) [19] . Primary antibodies used for immunofluorescence were anti-ubiquitin (Cell Signaling, P4D1, 1:100), anti-Mfn2 (Sigma, HPA030554, 1:100), anti-Tom20 (Santa Cruz Biotechnology, sc-11415, 1:2,000), and anti-Drp1 (BD Biosciences, 611,112, 1:500). Secondary antibody used were Alexa Fluor 647 goat anti-rabbit (Life Technologies, A21245, 1:1,000). Cell culture and transfections HeLa cells (ATCC, CCL-2) and COS-7 cells (CRL-1651) were both cultured in DMEM medium (Life technologies, 11,965) supplemented with 10% fetal bovine serum (Life Technologies, 10,437) and 1% penicillin/streptomycin (Life Technologies, 15,140), and maintained at 37 o C and 5% CO 2 . Cells were transfected with Lipofectamine 2000 (Life technologies, 11,668) based on the manufacturer’s protocol. CCCP (Sigma, C2759) was given at 10 μM. Wortmannin (Sigma, W1628) was given at 200 nM. MG-132 (Sigma, C2211) was given at 10 μM. Mdivi-1 (Enzo, BML-CM127) was given at 100 μM. Cells were stained with TMRE (Life Technologies, T-669) at 100 nM in cell medium for 20 min at 37 o C. Starvation-induced autophagy was triggered through incubating HeLa cells in EBSS (Life Technologies, 14,155) for 2 h. Live cell manipulation and imaging Light-assisted parkin-mediated mitophagy was performed on an Olympus FV1000 confocal microscope (60X, numerical aperture=1.2 water objective) equipped with a SIM scanner. HeLa cells were transferred into phenol-red-free medium for observation (Life Technologies; 31,053; containing fetal bovine serum and penicillin/streptomycin). Live HeLa cells were maintained under 37 o C and 5% CO 2 on the microscope for manipulation and observation (Tokai Hit, MIU-IBC). To achieve light-assisted parkin-mediated mitophagy, we point-scanned a 50-μW, 559-nm laser light through an ~10-μm × 10 μm region in a HeLa cell for a total of 30 s using Olympus FV1000’s tornado scanning. Movies were generated by imaging live cells at one frame every 2 min, with EBFP2-parkin detection using 405 nm excitation, EGFP-LC3B (as well as EGFP-Ub, AcGFP-sec61β and EGFP-DFCP1) detected using 488 nm excitation and KillerRed-dMito (as well as pTagRFP-DFCP1, mcherry-parkin and TMRE) detected with 559 nm excitation. A zero drift compensator module (Olympus) was used to correct sample drift in the z direction during live cell imaging. The images were not processed after acquisition. Immunofluorescence Ub, Mfn2 and Tom20 immunofluorescence were performed through the use of Alexa Fluor 647-labelled secondary antibodies (1:1,000) and detected with 635 nm excitation. HeLa cells were seeded on 35 mm MatTek gridded glass bottom dishes (P35G-2-14-C-GRID) and activated for mitophagy by 559 nm light. The cells were fixed with 2% paraformaldehyde from Electron Microscopy Sciences (15,711) for 10 min at room temperature, stained and imaged on a FV1000 Olympus confocal microscope. Drp1 immunofluorescence, on the other hand, was performed according to a previously published protocol [30] . How to cite this article: Yang, J.-Y. & Yang, W.Y. Bit-by-bit autophagic removal of parkin-labelled mitochondria. Nat. Commun. 4:2428 doi: 10.1038/ncomms3428 (2013).